Natural snowfall reveals large-scale flow structures in the wake of a 2.5-MW wind turbine To improve power production and structural reliability of wind turbines, there is a pressing need to understand how turbines interact with the atmospheric boundary layer. However, experimental techniques capable of quantifying or even qualitatively visualizing the large-scale turbulent flow structures around full-scale turbines do not exist today. Here we use snowflakes from a winter snowstorm as flow tracers to obtain velocity fields downwind of a 2.5-MW wind turbine in a sampling area of ~\n36 × 36 m 2 . The spatial and temporal resolutions of the measurements are sufficiently high to quantify the evolution of blade-generated coherent motions, such as the tip and trailing sheet vortices, identify their instability mechanisms and correlate them with turbine operation, control and performance. Our experiment provides an unprecedented in situ characterization of flow structures around utility-scale turbines, and yields significant insights into the Reynolds number similarity issues presented in wind energy applications. Laboratory and numerical studies of near-surface phenomena occurring in the atmospheric boundary layer (ABL) are severely constrained by the inability to reproduce the complexities of real-life atmospheric flow conditions and by an inherently limited range of spatial scales leading to enormous differences in Reynolds number. The challenge such limitations pose is best underscored in wind energy applications, where the rotor diameter of modern utility-scale wind turbines now reach above 100 m. Despite past and ongoing vigorous research [1] , [2] , [3] , [4] , the coupling of atmospheric flows with utility-scale turbines and multi-turbine wind power plants remain poorly understood, which contributes to sub-optimal performance at the plant scale with average power loss of 10–20% (refs 5 , 6 ). Our ability to gain such understanding is limited by the lack of experimental techniques able to quantify turbulent flows at the utility turbine scale. Current field measurement techniques provide only point velocity characterization (sonic anemometers) or velocity profiles (LiDAR and Sodar) at a coarse spatio-temporal resolution [7] , [8] , [9] . Particle image velocimetery (PIV), based on tracking the displacement of tracers in an illuminated flow field [10] , [11] , is the only measurement technique capable of obtaining planar velocity distributions with the spatio-temporal resolution required to study flow–structure interactions. However, PIV has only been applied, so far, to small-scale turbine models, from 0.1 m to a few metres in wind tunnel experiments [12] , [13] , [14] , [15] , [16] , [17] . One of the main obstacles to PIV implementation on a utility-scale turbine is the requirement to seed a large flow field (~\n100 m) with tracers uniformly and persistently distributed, in an environmentally benign, economic and non-intrusive fashion, which makes it almost impossible to use artificial seeding methods. In addition, the in situ PIV implementation is severely constrained by a number of adverse environmental conditions in the field such as the background daylight and large dynamic range of wind velocity and direction. Consequently, PIV has yet to be applied to areas larger than a few square metres [18] , [19] , [20] , which is at least one order of magnitude smaller than what is required to make an impact in wind energy research. Here we report super-large-scale PIV (SLPIV) measurements in the ABL behind a fully instrumented 2.5 MW wind turbine using natural snowflakes as tracer particles during a snowstorm in the early morning hours of 22 February 2013 in Rosemount, MN. In the experimental setup, a collimated 5-kW searchlight with specially designed reflecting optics is employed to generate a light sheet aligned with the mean wind direction for illuminating snow particles. The meteorological conditions contribute to optimal concentrations of snowflakes with good traceability and light-scattering capability, enabling flow visualization of coherent motions at elevations corresponding to the lower portion of the rotor behind the operating turbine. The SLPIV measurement uses a 25-MP high-resolution camera to resolve instantaneous trajectories of the snow particles in a sampling area of ~\n36 × 36 m 2 , within the region between 3 and 39 m above the ground. By cross-correlating time-consecutive images, the wind velocity distribution in the illumination plane is obtained at a spatial resolution of 0.44 m per vector at 30 Hz. The resolution is sufficient for quantifying the spatio-temporal evolution of large vortical structures induced by the rotating blades in the turbine wake. Taking advantage of the fully instrumented 2.5-MW turbine, we are able to synchronize the wake flow with operational and structural load data from the turbine to classify vortex structures in the turbine wake, examine their evolution, instabilities and mutual interactions, and correlate them with the operational control, power and structural loads of the turbine. Flow structures The advection patterns of snow particles within the light sheet elucidate the dynamics of unsteady vortical structures occurring in the turbine wake. The hallmark vortical structures are the three-dimensional vortex tubes shed at the blade tips, which are referred to as the tip vortices. As the turbine rotates, the tip vortices describe helical trajectories evolving with the turbine wake and intersect the light sheet at multiple streamwise locations, where vortex cores create voids in the snow particle seeding due to the centrifugal effect on the inertially driven snow particles ( Figs 1 and 2 ). Connected to, and positioned above each tip-vortex core, a vertical strip of low snowflake concentration is frequently observed ( Fig. 2f,g ). This signature is the footprint of trailing vortex sheets generated along the entire span of each blade. Compared with the tip vortices, these structures are less energetic and persistent, and have been visualized in the past only at small laboratory scales [21] . For most of the time during the observation period, the tip-vortex structures are advected downstream steadily, projecting a periodic streak pattern (or trail) of equally spaced voids ( Fig. 2g ). The starting angle φ of the streaklines, estimated by the initial trajectory of the vortex entering the imaging domain, indicates horizontal, upward or downward advection patterns of the tip vortices ( Fig. 2b–d ). We reason that unsteadiness in the incoming wind and the corresponding variation induced by the turbine control response result in the observed fluctuations of both φ and the spacing between adjacent voids. Although φ is loosely correlated with the blade pitch β ( φ has more fluctuations as compared with that of β ), steep downward advections with | φ |>15° are found to persistently occur around local minima of the blade pitch ( Fig. 2 ). The sharp variations in φ demonstrate the strong effect of the turbine operational control on the wake vortex dynamics and point to the possibility of developing advanced turbine controls for strategically manipulating wake dynamics to enable overall wind farm optimization. In our observation period, the tip-vortex streakline is predominately downward with a time-averaged angle < φ > of approximately −3°. The spacing between adjacent voids represents the helical pitch of tip-vortex spirals and, when decreased, tends to promote vortex interactions. Such interactions are observed only occasionally and involve two or more vortices with continual reduction in spacing, which then start to orbit around each other, ultimately merging into a new stronger vortex that rotates in the same direction with increased vortical circulation and size ( Fig. 2a ). More frequently, we observe events such as vortex collapse, visualized by a sudden homogenization of snow particle concentration in the collapsing vortex core and rapid vanishing of the characteristic void signature ( Fig. 2e ). This phenomenon, manifesting a drastic reduction of vortex strength, is a result of the breakdown of the trailing vortex sheets, which are needed to sustain the tip vortices [22] . The unsteadiness of the trailing sheets can quickly trigger tip-vortex instability and cause vortex core collapse and, subsequently, void disappearance. In fact, as observed in the experiment, the inception of vortex collapse resides at the transition from stable to unstable evolution of the trailing sheets ( Fig. 2e,f ). 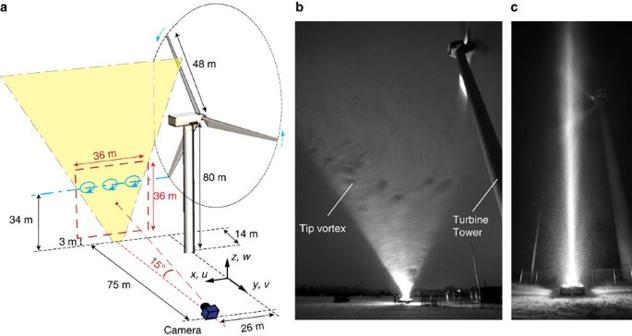Figure 1: The experimental setup for super-large-scale particle image velocimetry using natural snowfall. (a) A schematic of the setup during the deployment. (b) The frontal view and (c) the side view of the light sheet for illumination. Note thatFig. 1b,cwere taken using a Canon EOS T1i camera with wide-angle lens and subjected to image distortion. Figure 1: The experimental setup for super-large-scale particle image velocimetry using natural snowfall. ( a ) A schematic of the setup during the deployment. ( b ) The frontal view and ( c ) the side view of the light sheet for illumination. Note that Fig. 1b,c were taken using a Canon EOS T1i camera with wide-angle lens and subjected to image distortion. 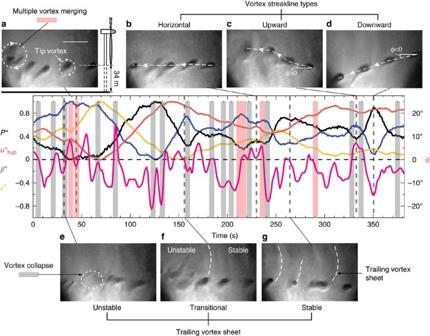Figure 2: A time sequence of near-wake vortical structures and incoming wind and turbine variables. The time sequence, from 3:12:18 am to 3:18:39 am on 22 February 2013, shows normalized turbine power (black line,P*), hub-height wind speed (red line,uhub*), blade pitch (blue line,β*), tip-speed ratio (orange line,λ*), and tip-votex streakline angle (magenta line,φ) defined in the insert panelscandd. The insert panelsa–gshow snapshots of tip vortices behind the turbine at different times in the time sequence. Red and grey shaded areas mark the occurrence of merging and collapsing vortices, respectively. Note thatP*=(P−<P>)/Pmax, wherePis the instantaneous power, <P> andPmaxare the mean and maximum power within the sampling period, respectively. The other variablesuhub*,β* andλ* are normalized in the same fashion. Scale bar, 10 m (a). Full size image Figure 2: A time sequence of near-wake vortical structures and incoming wind and turbine variables. The time sequence, from 3:12:18 am to 3:18:39 am on 22 February 2013, shows normalized turbine power (black line, P *), hub-height wind speed (red line, u hub *), blade pitch (blue line, β *), tip-speed ratio (orange line, λ *), and tip-votex streakline angle (magenta line, φ ) defined in the insert panels c and d . The insert panels a – g show snapshots of tip vortices behind the turbine at different times in the time sequence. Red and grey shaded areas mark the occurrence of merging and collapsing vortices, respectively. Note that P *=( P −< P >)/ P max , where P is the instantaneous power, < P > and P max are the mean and maximum power within the sampling period, respectively. The other variables u hub *, β * and λ * are normalized in the same fashion. Scale bar, 10 m ( a ). Full size image Overall, from Fig. 2 , we observe that the majority of vortex interaction events (80%, or 19 events out of 24 events in total), including merging and collapse, occur during the time spans of increasing tip-speed ratio λ . In addition, within the time span of increasing λ , vortex interaction events always occur in the vicinity of the local maxima of the blade pitch (in total seven local maxima, each one has one to three vortex interaction events in the neighbouring time spans). Some physical explanations are provided here to understand the trends described above. Increasing λ reduces the spacing between the consecutive vortices (the helical pitch) and may promote intense vortex–vortex interactions, which cause the onset of vortex merging to occur closer to the turbine [23] . Moreover, the coincidence of the vortex interaction events with local blade pitch maxima can be explained by the weakening of the tip-vortex strength due to turbine’s dynamic response to the incoming atmospheric turbulence. As illustrated in Fig. 2 , the local pitch maxima correspond to the local minima of power generation, which implies a reduction of tip-vortex strength as compared with neighbouring tip-vortex cores (more details are provided in our analysis of the correlation between tip-vortex circulation, blade pitch and angle of attack). Combined with the shifting of the vortex position due to the unsteady incoming wind, this perturbation on the vortex strength can lead to a rapid destabilization of wake vortical system and consequently to the grouping and merging events, as also evidenced in the numerical simulation by Delbende and Rossi [24] . Nevertheless, we do acknowledge that this is only a statistical, rather than an analytical description of what occurs in the wake, as not all the merging/collapse events satisfy the trend described above. These exceptions point to the conclusion that vortex interaction events may also be triggered by other factors that can influence the turbine wake and have not been considered in the present study. Such factors could include, for example, unsteadiness presented in the turbine operation and the unsteadiness and inhomogeneity of the near-blade turbulent flow induced by aeroelastic effects. Velocity distribution In Fig. 3a we present an instantaneous velocity field, after subtracting the snowflake settling velocity W s from the original vector field to demonstrate the quality of our velocity measurements. The resulting velocity distribution reveals the dominant wake-flow features [2] , [12] , such as the travelling vortex cores, the momentum entrainment between vortices (highlighted in Fig. 3c ), and the shear layer delineating the lower boundary between the turbine wake and the deflected incoming flow. To illustrate the features of the velocity profile presented in Fig. 3b , we introduce an artificially generated canonical log-law profile representing an undisturbed fully rough turbulent boundary layer. The profile is formulated as U + =( 1/κ ) ln(z/z o ), where U + is the mean streamwise velocity scaled by the friction velocity u *, von Kármán constant κ is chosen to be 0.41 and z/z o is the non-dimensional wall-normal height using the aerodynamic roughness length z o (ref. 25 ). By adjusting z o and u *, this profile, depicted as a dashed curve in Fig. 3b , fits (least square) the mean velocity in the range of 0.15< z / D <0.3. The fitting range is determined by observing the presence of the two distinct inflexion points at z / D =0.15 and 0.3 in mean velocity profile behind the turbine ( Fig. 3b ), respectively. Near the ground ( z / D <0.15), the velocity distribution shows an increase in velocity over the undisturbed fully rough turbulent boundary layer, suggesting a region of flow acceleration induced by the rotor-imposed blockage. At z / D =0.3, the velocity profile yields a maximum located below the lower tip, indicating a wake expansion angle of ~\n9° within ~\n1/3 of the rotor diameter from the turbine. Above the velocity maximum ( z / D >0.3), a sudden drop of velocity occurs, which is associated with the momentum deficit in the wake region. In the close-up view of the instantaneous flow field ( Fig. 3c ), the counter-clockwise rotating patterns of the fluctuating velocity vectors, marking each tip-vortex core, surround regions of low snow particle concentration (where snow SLPIV cannot be performed). These patterns confirm that the voids are indeed a strong signature of high-vorticity regions. Outside the voids, as discussed in the Traceability section in the Methods, considering a length scale l =2.6 m and velocity fluctuation u f ≈1.2 ms −1 associated with an individual vortex core, a representative time scale is given by τ f = l / u f ≈2.16 s. The corresponding Stokes number St=τ p /τ f ≈0.03 ( τ p is the particle response time) suggests that snow particles are deemed acceptable tracers for these large-scale motions in our sampling area ( Supplementary Methods ). 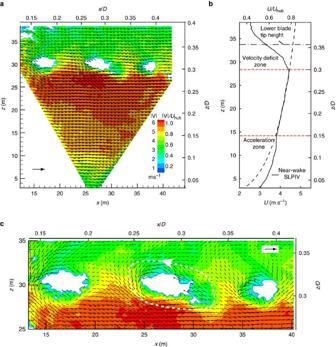Figure 3: Large-scale velocity field measurements behind 2.5 MW. (a) A sample of anx–zplane instantaneous velocity vector fields (with snowflake settling velocity removed) from SLPIV measurements superimposed with the contours of the velocity magnitude |V|. Non-dimensionalized velocity and locations are provided using mean wind speed at the hub height,Uhub=5.67 ms−1and rotor diameterD=96 m. (b) The time-averaged streamwise velocity profileUatx=26 m (the centre of the light sheet). The black dashed line is a canonical log-layer profile that fits the SLPIV mean velocity profile in the range of 0.15<z/D<0.3 to illustrate the velocity deficit and acceleration zone in the wake. (c) A close-up view of velocity field around tip-vortices. As illustrated inFig. 1, the origin ofxis at the centre of turbine tower and that ofzis at the ground. A Galilean translated vector field (u-0.9Uhub,v-0.1Uhub) is shown to visualize the counterclockwise rotation motion of vortices. The velocity vectors are skipped in 1:4 (a) and 1:2 (c) in bothxandzdirections for clarity. Scale bars, 6 ms−1(a) and 2 ms−1(c). Figure 3: Large-scale velocity field measurements behind 2.5 MW. ( a ) A sample of an x – z plane instantaneous velocity vector fields (with snowflake settling velocity removed) from SLPIV measurements superimposed with the contours of the velocity magnitude | V |. Non-dimensionalized velocity and locations are provided using mean wind speed at the hub height, U hub =5.67 ms −1 and rotor diameter D =96 m. ( b ) The time-averaged streamwise velocity profile U at x =26 m (the centre of the light sheet). The black dashed line is a canonical log-layer profile that fits the SLPIV mean velocity profile in the range of 0.15< z / D <0.3 to illustrate the velocity deficit and acceleration zone in the wake. ( c ) A close-up view of velocity field around tip-vortices. As illustrated in Fig. 1 , the origin of x is at the centre of turbine tower and that of z is at the ground. A Galilean translated vector field ( u -0.9 U hub , v -0.1 U hub ) is shown to visualize the counterclockwise rotation motion of vortices. The velocity vectors are skipped in 1:4 ( a ) and 1:2 ( c ) in both x and z directions for clarity. Scale bars, 6 ms −1 ( a ) and 2 ms −1 ( c ). Full size image Tip-vortex circulation Associated with each individual tip vortex, the circulation Γ, defined as the line integral of the velocity along a closed path enclosing the vortex core (such as the one marked in Fig. 3c ), can be quantified using SLPIV data ( Supplementary Fig. 1 and Supplementary Note 1 ). For each tip-vortex shed from a passing blade, the so-computed circulation remains relatively constant as the vortex is advected downstream within our sample area, which spans ~\n0.4 of the rotor diameter in the streamwise direction ( Supplementary Fig. 2 and Supplementary Note 1 ). This apparent low variance of the tip-vortex circulation in our imaging domain suggests that the roll-up process of trailing vortices is likely to be completed upstream of our measurement location. The tip-vortex circulation from SLPIV measurements can be compared with the averaged bound circulation on one blade estimated from the turbine power. The detailed analysis is provided in the Supplementary Note 2 . By assuming a constant bound circulation Γ along the blade, our analysis indicates that the mean tip-vortex circulation measured in our experiment captures ~\n39% of the blade-bound circulation derived from the power production. This percentage falls in within a range of reported values, that is, 35% to 90%, from laboratory experiments [26] and numerical simulations [27] . The incomplete capture of blade-bound circulation could be contributed by multiple sources such as the assumptions made during our calculations, the uncertainty involved in our measured circulation (details provided in Supplementary Note 1 ), the effect of blade geometry, and the effect of atmospheric turbulence on tip-vortex evolution. It is noteworthy that the high Reynolds number atmospheric turbulent flows and the large scale of the turbine do not seem to strongly affect the circulation capture by tip vortices on average, but may contribute significantly to the unsteadiness presented in the tip-vortex circulation as shown in the following section. Tip-vortex circulation versus turbine dynamics The synchronization of circulation measurements and turbine operational data (power output, blade pitch and foundation strain) allow us to expose the turbine’s dynamic control for power maximization and its structural response to unsteady wind conditions (flow–structure interaction). The circulation averaged over 5 s time intervals for each SLPIV run, <Γ>, correlates linearly with the turbine power averaged over the same time intervals, < P > ( Fig. 4a for five runs). However, within each SLPIV sequence, a significantly higher variability of Γ, among individual tip vortices passing across our sample area (four to five vortex core samples in one run), is observed when compared with the incoming wind velocity and power fluctuations in the same period ( Fig. 4a ). The circulation measurements, coupled to unsteady forces imposed on the blades, suggest that unsteadiness of the incoming flow is amplified through the interaction with the turbine, leading to a variety of coherent motions and interacting modes in the turbine wake ( Fig. 2 ). The reduced variability in the power output is primarily attributed to the spatial averaging effect in the conversion of the wind to a lift force, heterogeneity in the wind spanning the large rotor area and the large rotational inertia of the turbine rotor and drive train. The turbine control also contributes partially to the reduction of power fluctuations, specifically acting on the blade pitch β , to change the angle of attack α , and on the generator torque to control turbine rotational speed and thus to compensate for strong wind fluctuations. Hence, although α remains proportional to the tip-vortex circulation <Γ>, as expected in any conditions far from the aerodynamic stall, β is observed to decrease with increasing <Γ> ( Fig. 4b ). This trend is entirely consistent with the distinct out-of-phase correlation between β and <P> observed in Fig. 2 . The apparent strategy employed by the turbine controller to rapidly adjust the pitch in response to the approach wind velocity to maintain the generator speed dampens the unsteady fluctuations of the lift and thrust, and ultimately leads to a reduction of the power fluctuations. The condition of relatively constant generator speed, a characteristic of turbine controls in the region just above cut-in speed (noted as Region 1½ in Methods), implies that as the flow velocity increases, the instantaneous tip-speed ratio λ decreases ( Fig. 2 ). This interconnectedness suggests that as the circulation increases, due to an increase of the velocity, the angle between the relative wind velocity and the turbine axial direction θ , approximated by θ =arctan(1/ λ ), should also increase ( Fig. 4b ). Another key manifestation of flow–structure interaction is described here in terms of unsteady structural loading, as quantified by 20 strain gauges installed on the turbine foundation ( Supplementary Methods ). As the forces on the blades are translated into a tipping moment of the tower, a strong correlation between <Γ> and the turbine foundation strain < S> is expected, and this correlation is indeed confirmed by the results shown in Fig. 4c . 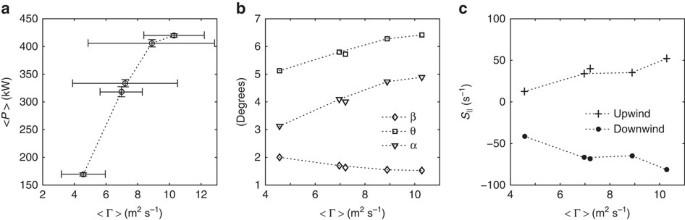Figure 4: Flow–turbine interactions evaluated during five independent super-large-scale particle image velocimetry runs. Circulation values are averaged along the vortex trajectory, for a variable number of vortices occurring within each 5 s long SLPIV run. (a) Measurements of mean turbine power <P>as a function of the mean circulation <Γ>; bars denote one standard deviation of power and circulation (varying for each tracked vortex within each SLPIV run), respectively. (b) Measurements of blade pitch angleβ, the angle between the relative wind velocity and the turbine axial direction θ and angle of attackα=θ−βas a function of <Γ>; (c) Measurements of mean strain along the wind direction at the tower foundation (positive values indicate stretching occurring at the downwind side, while negative values indicate compression at the upwind side). Figure 4: Flow–turbine interactions evaluated during five independent super-large-scale particle image velocimetry runs. Circulation values are averaged along the vortex trajectory, for a variable number of vortices occurring within each 5 s long SLPIV run. ( a ) Measurements of mean turbine power < P> as a function of the mean circulation <Γ > ; bars denote one standard deviation of power and circulation (varying for each tracked vortex within each SLPIV run), respectively. ( b ) Measurements of blade pitch angle β , the angle between the relative wind velocity and the turbine axial direction θ and angle of attack α = θ−β as a function of <Γ > ; ( c ) Measurements of mean strain along the wind direction at the tower foundation (positive values indicate stretching occurring at the downwind side, while negative values indicate compression at the upwind side). Full size image Our study presents the first measurements of unsteady flow structures behind a utility-scale turbine. The measurement technique, although constrained by specific weather conditions, allows us to make a number of novel contributions. First, SLPIV measurements within the turbine wake provide information of unsteady vertical structures, which can be correlated with turbine operations. The flow visualization using snowflakes evidences that the pairing and merging of two or three adjacent tip vortices and the collapse of vortices occur frequently within a half rotor diameter (that is, x / D =0.5) downstream of the turbine blades. Although the grouping of tip vortices has been observed in a number of prior studies [23] , [28] , it was reported to appear much farther downstream of the turbine when compared with that in our study. By correlating the visualized vortex structures with the synchronized turbine performance information, our experiment has shown some connection between the vortex interactions and subtle changes in the turbine operation. The early occurrence of such interactions, compared with the observations from laboratory experiments, is likely to be related to the significant unsteadiness that is uniquely presented in the turbulence of the ABL coupled with the subsequent response of the utility-scale turbine operation. As discussed in a number of recent studies [23] , [24] , [29] , the unsteadiness related to, for example, large perturbations due to incoming flow and rotor geometry, including inhomogeneities in the blade construction, can cause variation in initial vortex position and strength, and lead to a rapid destabilization of the vortex system and vortex interactions. The characteristics of vortex interaction observed in our study would imply a fast dissipation of wake structures and significantly different wake growth for a utility-scale turbine. For example, the ‘multi-step’ tip-vortex grouping mechanism reported in Felli et al . [28] and the interactions of tip vortices and the hub vortex [22] , [23] may manifest very differently for utility-scale turbines. All these issues pose important questions that will form the basis of future investigations, which will integrate the SLPIV technique with high-fidelity numerical simulations. Second, the current SLPIV measurement technique quantifies the instantaneous full-scale velocity field and tip-vortex circulation. Based on a general principle of PIV, our experiment is able to quantify the instantaneous turbulent flow fields at scales sufficiently large to make an impact on studying the aerodynamics around utility-scale turbines. The time-averaged flow field presents general features of near-wake flows. The circulation of neighbouring tip-vortex cores computed from instantaneous velocity fields shows considerably larger differences compared with the corresponding turbine power fluctuations. However, a circulation averaged over a 5 s interval (that is, a low-pass filtering) correlates linearly with turbine power generation and the percentage of blade-bound circulation captured by tip vortices is consistent with prior laboratory measurements [26] . Although the current flow quantification is limited up to lower portion of the rotor wake, the whole-field flow characterization around the turbine can be achieved through some hardware improvements, which include employing more powerful search lights and cameras with higher sensitivity. Other sophisticated data sets are envisioned in the near future by simultaneously measuring spatially resolved incoming and wake flows, as well as turbine performance and blade structural dynamics to achieve direct in situ characterization of flow–structure interactions. The approach in the present study can be employed to quantify turbulent flow fields in a substantial portion of the ABL, compared with previous PIV measurements in the ABL, which are typically within 2 m above the surface. This capability provides us an opportunity to investigate the organization of turbulent structures in high Reynolds number boundary layer flows, including problems such as the vertical extent and scaling of ramp-like structures and inner–outer layer interactions, forest and urban canopies focusing on shear penetration and dispersion processes, wake of buildings, bridges or other civil infrastructures for wind engineering applications. In addition, owing to the unique tracers used in our measurements, our technique can be naturally adapted to study a number of snow-related subjects for the cold climate regions, such as snow drift driven by large-scale turbulence, spatial variation of snowflake settling velocity, concentration and size distributions. Instrumented full-scale wind turbine The field experiment was performed at the University of Minnesota Eolos Wind Energy Research Field Station in Rosemount, MN ( Supplementary Fig. 3 and more details in Supplementary Methods ). The field station consists of a heavily instrumented 2.5-MW Clipper Liberty C96 wind turbine (hereafter referred to as the Eolos turbine) and a 130 m meteorological tower (hereafter referred to as the met tower). The Eolos turbine is a three-bladed, horizontal-axis, pitch-regulated, variable speed machine with a rotor diameter of 96 m mounted atop an 80 m tall supporting tower. The met tower ( Supplementary Fig. 4 ), located 160 m south of the turbine, is designed to characterize the local atmospheric meteorological conditions. Data from the field station is captured primarily with five synchronized sensor systems, including the standard turbine operational instrumentation, the rotor instrumentation for characterizing blade deformations, the turbine tower instrumentation for quantifying tower structural response, the foundation instrumentation and the met tower instrumentation, which comprises a number of wind velocity (sonic, cup and vane anemometers), temperature and humidity sensors installed at elevations ranging from 7 m to the highest point of the rotor, 129 m. The measurements from the five systems are sampled continuously 24 h a day and stored on backed up servers. Seeding mechanisms Natural snowfall provides particle seeding in a large sampling region for an extended period of time in an environmentally benign and non-intrusive fashion (details provided in Supplementary Methods ). In addition, snowflakes have strong light-scattering capability (especially side scattering) owing to their multi-facet crystalline structure, which lowers the illumination power required for particle imaging. Artificially generated snow was previously used for PIV measurement [30] . A major concern of seeding with snow particles is the limited traceability due to their inertial and gravitational effects associated with their relatively large density as compared with that of the air. In general, to trace a flow with time scale τ f , the traceability of particles can be characterized by the Stokes number, St=τ p /τ f , where τ p is the particle response time. The detailed discussion of the traceability of snowflakes in the presented experiment is provided in the Traceability section in the Methods and Supplementary Methods . Experimental setup The SLPIV setup ( Fig. 1 ) is composed of an optical assembly for illumination, a high-resolution imaging device and a data acquisition system. The optical assembly includes a 5-kW collimated searchlight (a divergence <0.3° and initial beam size of 300 mm in diameter) as a light source and a curved reflecting mirror for projecting a horizontal cylindrical beam into a vertical light sheet ( Supplementary Fig. 5 ). The sheet expansion angle is controlled by adjusting the mirror curvature. Supplementary Figure 6 illustrates a test of the light sheet generation at the Eolos site. By projecting the beam parallel to the ground, our measurements show that the beam diameter varies only from 300 to 600 mm in the first 100 m of its path, which ensures reasonably uniform thickness in both the vertical and horizontal span of our sampling area. The entire light system (including a 6-kW generator) is affixed to a trailer, providing good mobility for aligning the light sheet in the predominant wind direction as required for planar PIV measurements. The imaging device consists of a CMOS camera with a 50 mm f/1.2 Nikon macro imaging lens. The camera has a sensor of 5 K × 5 K pixels with 4.5 μm per pixel and captures up to 30 Hz at full sensor size. As the imaging device is tilted at an angle with respect to the ground as illustrated in Fig. 1 , a Scheimpflug adapter is employed for creating a slight angle between the lens plane and the camera sensor plane to achieve in-focus imaging of the entire sampling area. To calibrate our current setup, we first ensure that the tripod-mounted camera is levelled about its optical axis, which is aligned perpendicular to the light sheet. Next, we measure the tilt angle of the camera and its horizontal distance from the light sheet. Based on this information and the focal length of the imaging lens, we can correct the distortion resulting from the tilt imaging and determine the physical scale and location of the sampling area. Deployment The experiment (including both SLPIV measurements and video recording) was conducted from 2:00 to 3:30 am on 22 February 2013 during a snowstorm (details provided in Supplementary Methods , and a schematic of the deployment is presented in Supplementary Fig. 7 ). The weather and micrometeorological conditions during this period were obtained from the met tower and the Eolos turbine’s supervisory control and data acquisition system. The temperature measurements at all elevations below the turbine top-tip height stays between −6 °C and −7 °C with little fluctuations in time ( Supplementary Fig. 8a ). Similarly, the relative humidity remained nearly constant around 92%. However, the wind direction ( Supplementary Fig. 8b ) and speed ( Supplementary Fig. 8c ) were slowly changing in time. The predominant wind direction shifted from 54° (clockwise from north) at 2:00 am to 34° around 3:30 am, while the wind speed at the hub height dropped from ~\n8 to ~\n6 m s −1 . In this period, the bulk Richardson number, estimated from met tower measurements, is 0.06, indicating that the ABL was weakly stable. During the deployment, the Eolos turbine was operating in a transitional region between Region 1 and Region 2, namely, Region 1½. In this region, the blades continuously pitch to increase the aerodynamic lift, while applying minimal generator torque to allow the critical angular velocity ω to be reached. The light sheet was placed in the near-wake region of the Eolos turbine and aligned with the predominant wind direction around 2:00 am. ( Supplementary Fig. 7 ). The imaging device was then arranged perpendicular to the light sheet on the southern side. As illustrated in Fig. 1 , SLPIV measurement had a sampling area of ~\n36 × 36 m 2 , spanning 3–39 m above the ground. In this elevation span, the light sheet thickness varied from 320 to 420 mm according to the aforementioned tests. The camera was placed 75 m from the sampling plane in horizontal direction and tilted 15° with respect to the ground, resulting in a variation of pixel resolution 6.8–7.5 mm per pixel on the image sensor, which was accounted in the PIV vector calculation. The highest numerical aperture of 50 mm f/1.2 Nikon lens was used to achieve the maximum light reception, and the corresponding depth of field was calculated to be ~\n400 mm. Data processing The SLPIV vector fields were obtained by cross-correlating consecutive particle image pairs using an adaptive multi-pass algorithm in LaVision DaVis software. We used as an initial interrogation window of 256 × 256 pixels with 50% overlap and stepped down to a final window of 64 × 64 pixels. Consequently, the particle displacement in our recording period, ranging from 14 to 35 pixels, is <25% of initial interrogation window size, which satisfied the requirement of PIV cross-correlation algorithm. The selected interrogation window size also ensured sufficient particle density for valid PIV vector calculations ( Supplementary Fig. 9 and more details in Supplementary Methods ). The resulting spatial resolution dictated primarily by the interrogation window size was 0.44 m, which was close to the light sheet thickness and depth of field of the imaging system in the deployment. With 50% overlap of the interrogation windows, the vector spacing in the sampling field was 0.22 m. From 3:05 to 3:25 am, a total of eleven SLPIV runs were performed and used to obtain the near-wake mean velocity profile in Fig. 3 . Each run recorded 150 frames of 25-MP particle images and lasted 5 s. Five of these eleven data sets ( Supplementary Table 1 ) were synchronized with the turbine operation. The convection velocity for each individual vortex within the five data sets was calculated and used to determine the exact time at which each tip vortex was shed at the blade tip. The corresponding tip-vortex circulations were calculated ( Supplementary Table 2 ) with details provided in Supplementary Note 1 . This information is used to assess the correlation between tip-vortex circulations with turbine operation and performance ( Fig. 4 ). Traceability During our deployment, we measured the largest extension as the characteristic size of the snowflakes to be within the range of 1–3 mm by sampling the fresh snowflakes on the ground. In the acquired images for velocity vector field measurements, as illustrated in Supplementary Fig. 9a and Supplementary Movie 1 (enhanced snow particle image/movie samples), the snowflakes appeared 2–12 pixels in diameter. This discrepancy in imaged and the actual size of the snowflakes is attributed to several reasons such as the imaging magnification, the complex and multi-facet shape of snowflakes, the limited shutter speed and the illumination non-uniformity in elevation. To estimate the traceability of snowflakes, we approximated them as spherical particles. This assumption was employed in a number of prior studies on drag force analysis and settling velocity of snowflakes [31] . Based on the measured range of snowflake size, we assumed the snowflakes to be spheres of diameter d= 2 mm in the following calculation. Nevertheless, we acknowledge the fact that the snowflakes have much more complex morphology, the determination of which requires more sophisticated measurements. To evaluate τ p of snowflakes during our experiment, we first obtained an estimate of the settling velocity of snowflakes, found to be W s ≈0.65 ms −1 , using the spatio-temporal averaged vertical velocity from SLPIV measurements ( Supplementary Fig. 10 ). The measured W s ≈0.65 ms −1 is also relatively close to the results reported by Langleben [32] and Brandes et al . [33] for snow particles of similar size. Using the drag coefficient correction suggested by Crowe et al . [34] for particle Reynolds numbers outside of the Stokes regime, we obtained the same settling velocity for snowflakes of density ρ s ≈24.5 kg m −3 and diameter of d= 2 mm approximated as spherical particles. Using these calculated density and measured size, we calculated τ p = ρ s d 2 /[18 μ (1+0.15 Re p 0.687 )]≈0.07 s, where μ and Re p are the dynamic viscosity of the air and the particle Reynolds number, respectively [34] . Using the limiting case of the length scale l to be our SLPIV resolution (~\n0.44 m) and u f as the maximum value of the root-mean-squared streamwise velocity fluctuations in our sampling area (1.2 ms −1 ) resulted in τ f =l/u f ≈ 0.36 s representing the limiting timescale for our measurements. This time scale is equivalent to the turnover time of the smallest, but statistically representative energetic eddies that can be resolved with the spatial resolution of our measurements. The corresponding Stokes number, St= 0.19, quantifies the traceability of snowflakes along this limiting case eddy resolved in our sampling area (as the worst case scenario). The Stokes number drops in accordance with increasing scale of turbulent structures and decreasing velocity fluctuations, which suggests a substantial improvement of snow traceability for the large energetic turbulent motions. For instance, to resolve a turbulent eddy of ~\n2.6 m (characteristic scale of tip-vortex voids, details provided in Supplementary Note 1 ) with the same velocity scale above would yield St ≈0.03, in which case snow particles are deemed acceptable tracers. More detailed discussions of snowflake traceability are provided in in Supplementary Methods , including a comparison with a PIV tracer commonly used in the laboratory experiments such as olive oil droplets. Nevertheless, due to the complex and variable structure of snowflakes, we mainly rely on prior research [30] and our validation experiment (Toloui et al . [35] , briefly summarized in the following section and in Supplementary Methods ) to assess the quality of the measured velocity field using snowflake tracers. Uncertainty analysis and validation experiment The overall uncertainty of the SLPIV measurements is contributed by the calibration uncertainty, the uncertainties involved in PIV vector calculation and the convergence error for calculating mean velocity and turbulence statistics. As discussed in detail in Supplementary Methods , the uncertainties of the calibration process and PIV vector calculation for the current SLPIV experiment are estimated to be 0.057 and 0.045 ms −1 , respectively. The out-of-plane error is evaluated to be within the acceptable range for PIV measurements. The convergence error for mean velocity profile calculation is ~\n0.027 ms −1 . The measurement approach using the described experimental setup was validated through a separate set of study that focused on turbulent flow measurements in the ABL [35] . In this validation campaign, the SLPIV system was deployed in close proximity to the met tower at the Eolos wind energy research station, measuring turbulent flows in sampling area of ~\n22 m × 52 m, up to ~\n56 m above the ground. Comparing the mean velocity and in-plane turbulent kinetic energy from SLPIV and coincident sonic anemometers measurements at 10 and 30 m on the met tower, the results showed on average <3% and 8% difference, respectively ( Supplementary Fig. 11 ). The validation study also provided detailed uncertainty analysis of the measured mean velocity profile and turbulent statistics, which showed that the above discrepancy was within the measurement uncertainty of SLPIV. How to cite this article: Hong, J. et al . Natural snowfall reveals large-scale flow structures in the wake of a 2.5-MW wind turbine. Nat. Commun. 5:4216 doi: 10.1038/ncomms5216 (2014).